Three-dimensional eukaryotic genomic organization is strongly correlated with codon usage expression and function It has been shown that the distribution of genes in eukaryotic genomes is not random; however, formerly reported relations between gene function and genomic organization were relatively weak. Previous studies have demonstrated that codon usage bias is related to all stages of gene expression and to protein function. Here we apply a novel tool for assessing functional relatedness, codon usage frequency similarity (CUFS), which measures similarity between genes in terms of codon and amino acid usage. By analyzing chromosome conformation capture data, describing the three-dimensional (3D) conformation of the DNA, we show that the functional similarity between genes captured by CUFS is directly and very strongly correlated with their 3D distance in Saccharomyces cerevisiae , Schizosaccharomyces pombe , Arabidopsis thaliana , mouse and human. This emphasizes the importance of three-dimensional genomic localization in eukaryotes and indicates that codon usage is tightly linked to genome architecture. Understanding the importance of genome architecture, the arrangement of genes within the genome and how this organization evolved has been intensively studied in recent years. It has become evident that the genomic architecture and thus the three-dimensional organization of genes in the genome are far from random [1] , [2] , [3] , [4] . It is well-established that genomes tend to have specific conformations, typical organization during different steps of the cell cycle and specific regions that are more efficiently transcribed [5] , [6] , [7] , [8] . Thus, many previous studies have suggested that constraints on gene expression and function have shaped the organization of genes in the genome. Due to lack of appropriate data related to the three-dimensional genomic organization, earlier studies considered the one-dimensional (linear) organization of genomes, and many of them emphasized the higher levels of genomic organization in prokaryotes compared with eukaryotes; for example, it is known that prokaryotes (unlike most eukaryotes) tend to contain operons of co-transcribed genes with related function [9] . Recently, a new experimental approach for studying the three-dimensional (3D) architecture of genomes, Chromosome Conformation Capture (3C) [10] , has enabled far more accurate characterization of genomic spatial organization. Indeed, 3C and its derivative hi-throughput variants (such as Hi-C [11] ) have yielded a much improved picture of the 3D architecture of genomes in recent years. The general protocol consists of the following steps: cross-linking of interacting DNA segments; digestion using a restriction enzyme such as HindIII; circularization by ligation—so that a large portion of the products include a ring with fragments from both ends of the cross-linked interacting DNA pair; and finally, reversal of the cross links. The next steps differ from method to method, and ultimately conclude with the sequencing and mapping of DNA fragments to their original positions on the chromosomes [10] , [11] , [12] , [13] . Specifically, such whole-genome contact maps have recently been published, including those of Homo sapiens (HS) [11] , Saccharomyces cerevisiae (SC) [12] , Schizosaccharomyces pombe (SP) [13] , Caulobacter crescentus [14] , Drosophila melanogaster [15] , Mus musculus (MM) [16] , Arabidopsis thaliana (AT) [17] and Plasmodium falciparum [18] . In addition to an enhanced view of the global genome architecture of the aforementioned organisms, these studies revealed some associations with functional properties of genes and other genomic features. For example, it was shown that centromeres, telomeres, transfer RNAs (tRNAs), chromosomal breakpoints and early replication origins in SC [12] tend to be co-localized. In SP, significant co-localization was shown for highly expressed genes, G2 co-regulated genes and some genes that were functionally related, according to gene ontology (GO) terms [13] . In humans, clustering of contact maps revealed a transcriptionally active, GC-rich cluster, alongside two GC-poor clusters with low transcription activity [6] , [11] . Moreover, recently a correlation has been suggested between transcription factor network models and distances between average chromosome positions in human cells [19] . A series of studies further reported the co-localization of each of the following groups in SC: cohesin binding sites [20] , co-expressed genes, some identified GO terms [21] and gene targets of the same transcription factor [22] . Recently, an analysis of the genomic organization of the unique P. falciparum parasite throughout its cell cycle confirmed a relation between chromosome conformation and gene expression [18] . Here we hypothesize that genes with shared function and expression levels will tend to be close in 3D space, which will facilitate their co-transcription by shared transcription factors and optimize chromatin remodelling. We suggest that the reason that the previously observed association between gene function and 3D genomic organization was relatively weak is on account of the measures used to assess gene functional similarity, that were not sufficiently sensitive. Here we apply a novel unbiased measure of gene function/expression similarity, based on the similarity in codon distribution between genes, to reveal a strong link between 3D localization and function in eukaryotes. The results presented here provide the first global analysis in single-gene resolution of the spatial organization in multiple eukaryotes. The codon usage frequency similarity as functional distance Previous studies reported various significant, yet relatively weak associations between the 3D genomic distance (3DGD) and various specific functional aspects. These weak associations can be attributed to five major reasons that are not mutually exclusive: first, all the databases related to gene function are highly partial; there are genes with profuse information regarding their function, while others are yet to be explored, or include partial and sometimes erroneous data. Second, all large scale experimental biological data include various sources of noise and bias; third, most of the information related to functional attributes is discrete or binary (for example, the gene has/does not have a certain function or attribute) and not continuous. Fourth, functions are often subjectively defined, and are based on the specific experience and knowledge of the researcher(s) reporting them, and on the nomenclature that they prefer to use. Finally, most approaches used in the context of functional similarities are not metrics in the strict sense, and can be hard to quantify and interpret. Here we propose a novel measure of functional and expression similarity between genes, the codon usage frequency similarity (CUFS), which is based on the frequency of all codons within genes, and thus also reflects similarities in amino acid usage. We utilize this measure to study the relation between functional and genomic 3D distance. The measure is based on the Endres–Schindelin metric [23] , which in turn is based on the Kullback–Leibler divergence for information gain—a measure widely used in the information theory field for comparing probability distributions (see Methods). Briefly, given a pair of open reading frames (ORFs) the CUFS returns a distance estimation that is related to the codon content and distribution in the two genes: the more similar genes are in terms of the frequency of their codons (and amino acids), the shorter the distance between them. CUFS can thus be computed for any pair of genes (based solely on their genomic sequences), is not based on subjective definitions, is expected to be less biased/noisy than other large scale genomic data (sequencing errors are relatively rare in comparison to noise/bias in measurements of gene expression and physical interactions), and is a continuous measure that may be considered a metric. Most importantly, CUFS clearly measures various aspects of functional similarity and can serve as a proxy for such similarity: First, it incorporates similarity in amino acid content between gene pairs, which is a property strongly connected to function [24] . Second, as can be seen in Supplementary Fig. 1 , CUFS is strongly related to various gene features, among them gene expression level, protein–protein interaction (PPI) graph distance and GO terminology distance, as can be expected from a measure of functional similarity (technical details regarding how these measures were computed appear in the Methods section). Finally, it is clear that codon bias is related to various aspects of gene expression regulation [25] , [26] , [27] , [28] , [29] , which should be related, at least partially, to gene function in various ways [30] . For example, recently it was shown that non-optimal codon bias, in terms of adaptation to the tRNA pool, is a mechanism to achieve circadian clock [31] , [32] . Furthermore, a recent study suggested that transcription factors located within exons provide additional evolutionary constraints that shape the codon usage bias (CUB) of genes [33] . It is important to emphasize that despite the fact that CUFS is known to be also related to post-transcriptional aspects of gene expression, and that genomic organization of genes may be related to transcription optimization, the strong relation between CUFS and functionality gives rise to a strong correlation with 3DGD between genes, as reported in the following sections. For example (see Fig. 1 ), one aspect of genomic organization and gene function is expression levels; genes with similar transcriptional levels are expected to be clustered in the 3D genomic organization [5] , [6] , [7] , [8] , [13] ; for instance, highly expressed genes are expected to be clustered in regions that enable more efficient transcription and/or better transport of the messenger RNA (mRNA) out of the nucleus ( Fig. 1a ); we also expect that genes with similar translation levels (that tend to have similar transcription levels, see [34] ) will have similar CUFS; for example, highly expressed genes usually undergo stronger selection for codons that are more adapted to the intracellular tRNA pool [27] ( Fig. 1b ); cumulatively, these aspects contribute to the correlation between CUFS and 3DGD ( Fig. 1c ). To summarize our objective: CUFS is shown to be strongly connected to and a good proxy of gene expression and function ( Fig. 1d ). We aim to show that the function and expression of genes are strongly related to their genomic organization; if this is indeed true, we expect a strong relation, and that evolution will shape CUFS and 3DGD in a coordinated way. Indeed we observe that there is a strong correlation between function and expression of genes, as reflected in CUFS, and their 3D genomic organization. 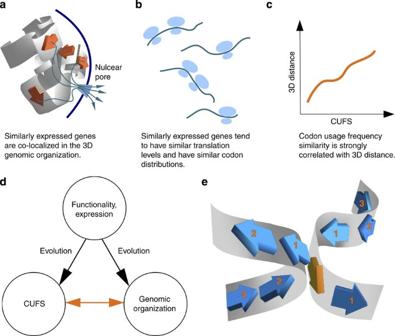Figure 1: General research approach. (a) An illustration of examples of hypothetical evolutionary processes that contribute to the observed strong correlation of CUFS and genomic distance. Genes with similar transcription levels are expected to be clustered in the 3D genomic organization (for example, highly expressed genes are clustered in efficiently transcribed and/or transport regions as these may be a more accessible part of the DNA, and/or in regions that tend to be closer to the nuclear pore), and thus are inclined to be closer in the 3D genomic organization. (b) We expect that genes with similar translation levels (that tend to have similar transcription levels) will have similar CUB; for example, highly expressed genes usually undergo stronger selection for codons that are more adapted to the intracellular tRNA pool to improve translation efficiency27, and thus have more similar CUB. (c) Eventually, a correlation between CUFS and 3D genomic distance is observed, although CUFS is related to translation and not only to transcription. (d) Plan of study: CUFS is known to be related and thus to evolve with gene expression and functionality (left arrow); we want to show that genes functionality and expression are strongly related to their genomic organization (right arrow); thus, by showing that there is a strong relation and adaptation between CUFS and 3D genomic distance (orange arrow), we actually show that there is strong correlation between the functionality and expression of genes and their 3D genomic organization. (e) Representation of the data. The diagram displays a single measured interaction between two DNA fragments, based on Hi-C data. Each arrow is a protein-coding gene, as well as a node on the graph. The interaction was mapped to be between the two nodes (arrows) closest to the point of interaction. The orange arrow is a reference node for all distances in the diagram (denoted in orange numbers on each node); see further details in Methods section. Figure 1: General research approach. ( a ) An illustration of examples of hypothetical evolutionary processes that contribute to the observed strong correlation of CUFS and genomic distance. Genes with similar transcription levels are expected to be clustered in the 3D genomic organization (for example, highly expressed genes are clustered in efficiently transcribed and/or transport regions as these may be a more accessible part of the DNA, and/or in regions that tend to be closer to the nuclear pore), and thus are inclined to be closer in the 3D genomic organization. ( b ) We expect that genes with similar translation levels (that tend to have similar transcription levels) will have similar CUB; for example, highly expressed genes usually undergo stronger selection for codons that are more adapted to the intracellular tRNA pool to improve translation efficiency [27] , and thus have more similar CUB. ( c ) Eventually, a correlation between CUFS and 3D genomic distance is observed, although CUFS is related to translation and not only to transcription. ( d ) Plan of study: CUFS is known to be related and thus to evolve with gene expression and functionality (left arrow); we want to show that genes functionality and expression are strongly related to their genomic organization (right arrow); thus, by showing that there is a strong relation and adaptation between CUFS and 3D genomic distance (orange arrow), we actually show that there is strong correlation between the functionality and expression of genes and their 3D genomic organization. ( e ) Representation of the data. The diagram displays a single measured interaction between two DNA fragments, based on Hi-C data. Each arrow is a protein-coding gene, as well as a node on the graph. The interaction was mapped to be between the two nodes (arrows) closest to the point of interaction. The orange arrow is a reference node for all distances in the diagram (denoted in orange numbers on each node); see further details in Methods section. Full size image A strong correlation between 3DGD and CUFS In this work, we focus on the preeminently studied mammalian species—MM and HS, known to have diverged 65 million years ago [35] , as well as a fungal pair—SC and SP, two yeast species known to have diverged 350–1,000 million years ago [36] , and a single plant—AT. For this purpose, we analyzed recently published whole-genome Hi-C contact maps [11] , [12] , [13] , [16] , [17] at single-gene resolution (see also Supplementary Table 1 ). We utilized the contact maps from these studies to construct a network/graph with protein-coding genes as nodes and edges depicting contacts between segments in the vicinity of these genes (generated by the Hi-C approach). To this end, each gene was mapped to its closest Hi-C segment, measured from the centre of the gene (see Methods). This graph representation can be used to compute a measure of 3DGD between each pair of genes; for example, genes corresponding to segments with Hi-C contacts are at the lowest distance rank (1 unit); pairs of genes that are not directly connected but are both connected to the same third gene have a larger distance rank (2 units), and so forth (see Fig. 1e ). It is important to mention that this graph representation was selected after a careful evaluation process that demonstrated that it is more robust to noise/biases in the Hi-C data than alternative representations. For example, we constructed a non-binary, weighted graph/network based on the same data as the binary graph, where edges’ values represent distances that are a function of the Hi-C reads (see Supplementary Methods ). We compared the genomic distances on both graphs to two previously published 3D models of complete fungi genomes [12] , [13] (see Supplementary Methods ). The two models were constructed by solving a polymer folding problem, employing non-linear constrained optimization obtained from the same Hi-C experiments our analyses are based upon. It is evident that the binary graph is more consistent with the 3D models than the weighted graph (SC: r =0.56 versus r =0.21, respectively, P <10 −323 , two-tailed t -test; SP: r =0.22 versus r =0.05, respectively, P <10 −323 ; Supplementary Fig. 2 ). We also tested the robustness of the models to noise, by generating pairs of models from partial sets of data and examined their consistency with each other. The binary model was considerably more consistent ( r =0.91, average on five organisms) than either the weighted model ( r =0.55) or raw Hi-C reads ( r =0.40; Supplementary Fig. 2 ). Intuitively, the relative robustness of the method may be related to the fact that all the edges (and thus all Hi-C 3D distances) are based only on very reliable Hi-C relations, and that the binary discretization filters noise/biases. 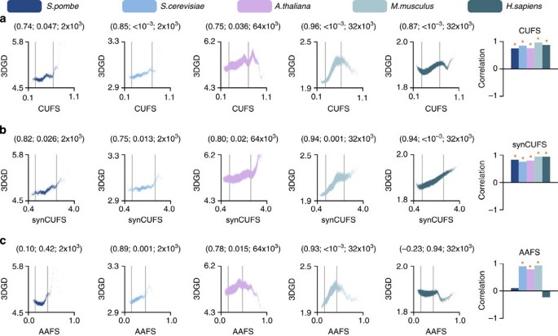Figure 2: Correlation between CUFS and 3D genomic distance. (a) Scatter plots of 3D genomic distance (3DGD) versus CUFS for the five organisms, (2 × 103points for fungi, 64 × 103forA. thalianaand 32 × 103for mammals on account of their genome size). Spearman’s rank correlation, P3DPvalues and number of points are reported in parentheses above each plot in this order. Vertical markers denote the top/bottom 5% of values, so that 90% are contained within them. Bars denote Spearman’s rank correlation coefficient,Pvalues were computed using the cyclic chromosome shift model (P3D, 1,000 samples drawn); stars mark significant correlations (P3D<0.05). (b) Scatter plots of 3DGD versus synonymous codon usage frequency similarity (synCUFS). (c) Scatter plots of 3DGD versus amino acid frequency similarity (AAFS). Next, we divided all gene pairs obtained in this manner into n bins with similar CUFS values; the number of bins ( n =2 × 10 3 in fungi, n =32 × 10 3 in mammals and n =64 × 10 3 in AT) was adjusted to account for the increase in genome size (see also Supplementary Table 2 ). The following step was to compute the mean genomic distance between gene pairs in each bin, and obtain the Spearman correlation between the 3DGD and CUFS ( Fig. 2a ). It should be noted that the large number of pair-distance values (~17 × 10 6 , for example, in SC) enables us to use a large n for binning, while reducing biological noise through averaging. Figure 2: Correlation between CUFS and 3D genomic distance. ( a ) Scatter plots of 3D genomic distance (3DGD) versus CUFS for the five organisms, (2 × 10 3 points for fungi, 64 × 10 3 for A. thaliana and 32 × 10 3 for mammals on account of their genome size). Spearman’s rank correlation, P 3D P values and number of points are reported in parentheses above each plot in this order. Vertical markers denote the top/bottom 5% of values, so that 90% are contained within them. Bars denote Spearman’s rank correlation coefficient, P values were computed using the cyclic chromosome shift model (P 3D , 1,000 samples drawn); stars mark significant correlations (P 3D <0.05). ( b ) Scatter plots of 3DGD versus synonymous codon usage frequency similarity (synCUFS). ( c ) Scatter plots of 3DGD versus amino acid frequency similarity (AAFS). Full size image The correlation observed between CUFS and 3DGD ( Fig. 2a ) was very high for all five organisms: SP ( r =0.74; P <10 −323 ; n =2 × 10 3 , two-tailed t -test), SC ( r =0.85; P <10 −323 ; n =2 × 10 3 ), AT ( r =0.75, P <10 −323 ; n =64 × 10 3 ), MM ( r =0.96; P <10 −323 ; n =32 × 10 3 ) and HS ( r =0.87; P <10 −323 ; n =32 × 10 3 ). The differences between the correlations we obtained in the specific organisms could reflect not only biological properties, but also aspects related to the different experimental procedures employed when the data were acquired (see Methods). As an example, correlations in mouse could be higher due to the better quality of this data set (see Supplementary Note 1 ). Despite the strong correlations, we observed occasional non-monotonic regions at the extreme ends of the plots, related to a small fraction of the genes and discussed in Supplementary Note 2 . While we could also obtain significant correlations between 3DGD and other gene sequence features, such as GC content ( Supplementary Fig. 3 ), as well as functional experimental measurements ( Supplementary Fig. 4 ), CUFS outperformed these regardless of the number of bins used when averaging across the five organisms ( Supplementary Fig. 5 ). Moreover, the P values of the correlations for different bin numbers and for raw data are identical. To better understand the different components that compose CUFS, we studied the correlations of synonymous codon usage (synCUFS, Fig. 2b ), amino acid frequencies (AAFS, Fig. 2c ), and GC content in the 3rd codon position (GC3, Supplementary Fig. 3 ). It is evident that the relation between synCUFS and 3DGD is very similar to the one observed for CUFS, with the former being more monotone in the higher eukaryotes (plant and mammals). AAFS, on the other hand, displays a non-monotonicity in the form of a tail of decreasing 3D distances in the higher eukaryotes. The correlation observed for AAFS is also more varied between organisms. CUFS is more strongly correlated than synCUFS in SC and mouse, and more strongly correlated than AAFS in SP, mouse and human. Plant and mammals also show a decreasing 3DGD profile with the average GC3 content of gene pairs, unlike the fungi. When studying the similarity in GC3 content between pairs of genes (see Methods), we observe positive correlations similar to CUFS, with the exception of AT. This was expected, as GC3 content and codon usage are known to be correlated. It should be noted, that both synonymous and non-synonymous features of the ORF are known to be related to protein function and expression [31] , [32] , [33] , [37] , [38] , [39] , [40] , [41] ; thus, our choice of CUFS attempts to capture and integrate as many as possible of the underlying signals in the coding sequence, for a better representation of the functional interactions between genes. Genomic organization extends beyond linear gene order To demonstrate that the correlations we obtained are not merely the product of 1D gene organization along the chromosomes, but that the chromosomal 3D location and the interaction between chromosomes also play a role, we employed a novel statistical test—P 3D . This test includes a conservative empirical null model—cyclic chromosome shift (see Fig. 3 and Methods). The randomized model preserves two major properties in genomic space: (a) The spatial conformation of the chromosomes (that is, graph edges) is left intact, while the genes rotate around it ( Fig. 3a ); (b) The linear adjacency between genes along the chromosomes is preserved. Thus, if the correlation observed between CUFS and 3DGD is significantly higher than that expected by the cyclic chromosome shift random model, we can reject the hypothesis that the observed correlation between function and 3DGD is mainly due to linear (1D) distances along chromosomes. Indeed, as can be seen in Fig. 3b,c P 3D <10 −3 in SC and in HS (1,000 samples drawn). P 3D values for other correlations are similar and appear in Fig. 2 . 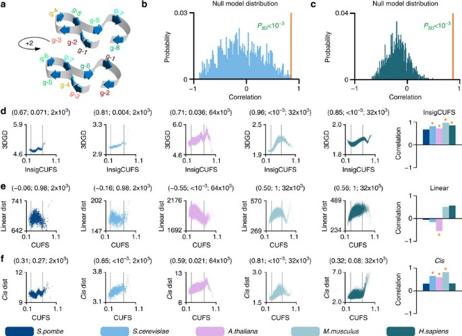Figure 3: Null model and linear organization. (a) A diagram of cyclic chromosome shift, depicting a shift two places counter-clockwise. While the spatial arrangement of nodes (arrows/genes) is preserved, as well as the adjacency between nodes, the labels (depicted by colours) are shifted two places around the chromosome (see details in Methods). (b) Distribution of Spearman’s correlation coefficient for 3D genomic distance (3DGD) versus CUFS when drawing 1,000 samples from the null model (seea), forS. cerevisiaeand (c)H. sapiens. The orange line represents the correlation result on experimental data and the adjacent label denotes the P3Dvalue for it. (d) InsigCUFS (see definition in the main text) shows the correlation obtained for CUFS versus 3DGD when excluding sets of genes that are significantly co-localized in a single Hi-C bin. Strong correlation is retained, thus the correlation observed for CUFS is not due to the resolution of the Hi-C maps. Spearman’s rank correlation, P3DPvalues and number of points are reported in parentheses above each plot in this order. Bars denote Spearman’s rank correlation coefficient,Pvalues were computed using the cyclic chromosome shift model (P3D, 1,000 samples drawn); stars mark significant correlations (P3D<0.05). (e) Correlation between CUFS and distances on a linear graph (measured in number of genes), showing reduced and insignificant correlation, as expected from P3D. (f) Correlation between CUFS and distances on a graph containing onlycis-chromosomal edges, showing significant correlations, but considerably lower than that for the complete model. Figure 3: Null model and linear organization. ( a ) A diagram of cyclic chromosome shift, depicting a shift two places counter-clockwise. While the spatial arrangement of nodes (arrows/genes) is preserved, as well as the adjacency between nodes, the labels (depicted by colours) are shifted two places around the chromosome (see details in Methods). ( b ) Distribution of Spearman’s correlation coefficient for 3D genomic distance (3DGD) versus CUFS when drawing 1,000 samples from the null model (see a ), for S. cerevisiae and ( c ) H. sapiens . The orange line represents the correlation result on experimental data and the adjacent label denotes the P 3D value for it. ( d ) InsigCUFS (see definition in the main text) shows the correlation obtained for CUFS versus 3DGD when excluding sets of genes that are significantly co-localized in a single Hi-C bin. Strong correlation is retained, thus the correlation observed for CUFS is not due to the resolution of the Hi-C maps. Spearman’s rank correlation, P 3D P values and number of points are reported in parentheses above each plot in this order. Bars denote Spearman’s rank correlation coefficient, P values were computed using the cyclic chromosome shift model (P 3D , 1,000 samples drawn); stars mark significant correlations (P 3D <0.05). ( e ) Correlation between CUFS and distances on a linear graph (measured in number of genes), showing reduced and insignificant correlation, as expected from P 3D . ( f ) Correlation between CUFS and distances on a graph containing only cis -chromosomal edges, showing significant correlations, but considerably lower than that for the complete model. Full size image We performed an additional control, testing for adjacent genes that were associated with the same Hi-C bin when constructing our model, and may contain significantly low CUFS (when compared with samples from the cyclic shift model). Such co-localized CUFS clusters may add bias to the reported correlation with 3DGD (through adjacent genes being assigned with identical Hi-C edges), but will not be controlled for by cyclic chromosome shift. This scenario becomes more plausible as the resolution of the Hi-C maps decreases and the number of Hi-C bins assigned with multiple genes increases. However, only a small percentage (1–5%) of Hi-C bins was found to have significant CUFS (P 3D <0.05, SP: 34 bins; SC: 49 bins; AT: 112 bins; MM: 281 bins; HS: 105 bins). We confirmed that genes associated with these Hi-C bins do not contribute more than expected to the correlation with 3DGD, by excluding them when computing the correlation (InsigCUFS, see Fig. 3d ) and observing that the correlation is retained (SP: r =0.67; P <10 −323 ; P 3D =0.071; n =2 × 10 3 ; SC: r =0.81; P <10 −323 ; P 3D =0.004; n =2 × 10 3 ; AT: r =0.71; P <10 −323 ; P 3D =0.036; n =64 × 10 3 ; MM: r =0.96; P <10 −323 ; P 3D <10 −3 ; n =32 × 10 3 ; HS: r =0.85; P <10 −323 ; P 3D <10 −3 ; n =32 × 10 3 ). It should be noted that the reported correlations with 3DGD are significantly higher than the ones obtained when considering only linear organization (SP: r =−0.06; P =0.007; P 3D =0.985; n =2 × 10 3 ; SC: r =−0.16; P =1.7 × 10 −12 ; P 3D =0.982; n =2 × 10 3 ; AT: r =−0.55; P <10 −323 ; P 3D <10 3 ; n =64 × 10 3 ; MM: r =0.50; P <10 −323 ; P 3D =1.00; n =32 × 10 3 ; HS: r =0.56; P <10 −323 ; P 3D =1.00; n =32 × 10 3 ; Fig. 3e , see the Supplementary Methods ). There is a non-significant, positive correlation in mammals, no correlation for yeast and a negative correlation in AT. The correlations obtained when considering only cis- Hi-C contacts are considerably higher ( Fig. 3f ), but still fall short of the correlation for the complete model (incorporating trans - as well as cis - contacts). Thus, we conclude that the observed organization of genes based on their function is strongly connected to the 3D conformation and organization of the chromosomes. CUFS correlates more strongly with 3DGD than CUB measures To better understand the role of codon usage as reflected in the 3D genomic organization, we performed a similar analysis to the one presented in the previous sections while employing different definitions of CUB: the codon adaptation index [42] (CAI); the tRNA adaptation index [29] (tAI); the background corrected effective number of codons [43] (bcENC); the codon deviation coefficient [44] (CDC) and the relative codon bias [45] (RCB) index ( Fig. 4 and Supplementary Fig. 6 ). The aforementioned indices measure the CUB of a single gene relative to a reference (a set of highly expressed genes [42] , the tRNA pool [29] or mutation bias [43] , [44] , [45] ). Thus, their definitions need to be extended to describe gene-pair interactions and to enable comparison with 3DGD and with CUFS, which inherently describe the relation between pairs of genes. One approach to do so could be to study the average bias of pairs of genes ( Fig. 4 , details in Methods). We observed that both the CAI and tAI show negative correlations with 3DGD, implying that highly adapted/biased genes—that also tend to be highly expressed—are closer spatially and vice versa . Interestingly, although CUB indices are typically poor predictors of gene expression in mammals, the correlation with 3DGD is stronger in human and mouse than in the fungi or plant. Another approach to extending the definition of these indices is to study the normalized index distance between pairs of genes ( Supplementary Fig. 6 , details in Methods). Since similarly biased genes tend to have similar expression levels, and since we hypothesize that genes with similar expression levels tend to be co-localized spatially, we expect to see a positive correlation between CUB similarities and 3DGD, which is indeed the case. It should be noted that this distance definition may place genes that are biased differently, but to a similar extent, in close proximity, as opposed to CUFS (they are 1D distances, instead of 64D distance, and consequently information is lost). We observed that this distance definition was in general positively correlated with 3DGD. Specifically, CDC similarity and RCB similarity resulted in positive correlations in all organisms, albeit lower than those seen for CUFS and spanned a narrower range of 3DGD values. 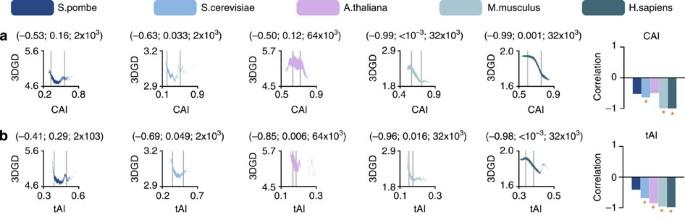Figure 4: Comparison of CUB measures. (a) Scatter plots of 3D genomic distance (3DGD) versus CAI (average of gene pairs) for the five organisms. Spearman’s rank correlation, P3DPvalues and number of points are reported in parentheses above each plot in this order. Vertical markers denote the top/bottom 5% of values, so that 90% are contained within them. Bars denote Spearman’s rank correlation coefficient,Pvalues were computed using the cyclic chromosome shift model (P3D, 1,000 samples drawn); stars mark significant correlations (P3D<0.05). (b) Scatter plots of 3DGD versus tAI (average of gene pairs). Figure 4: Comparison of CUB measures. ( a ) Scatter plots of 3D genomic distance (3DGD) versus CAI (average of gene pairs) for the five organisms. Spearman’s rank correlation, P 3D P values and number of points are reported in parentheses above each plot in this order. Vertical markers denote the top/bottom 5% of values, so that 90% are contained within them. Bars denote Spearman’s rank correlation coefficient, P values were computed using the cyclic chromosome shift model (P 3D , 1,000 samples drawn); stars mark significant correlations (P 3D <0.05). ( b ) Scatter plots of 3DGD versus tAI (average of gene pairs). Full size image Function–location relationships are conserved in evolution To better understand the evolutionary properties of function–location relationships, we focused on the subset of genes that had orthologues both in SC and SP (3,367 orthologue families; see Methods), as well as orthologues in human and mouse (15,832 orthologue families). Notably, the CUFS between gene pairs in different organisms was highly conserved in both organism groups (HS-versus-MM : r =1.0; P <10 −323 ; n =32 × 10 3 ; SC-versus-SP : r =1.0; P <10 −323 ; n =2 × 10 3 , two-tailed t -test). In addition, the 3DGD between gene pairs in different organisms also showed significant correlation (HS-versus-MM : r =0.57; P <10 −323 ; n =32 × 10 3 ; SC-versus-SP : r =0.13; P =5.7 × 10 −9 ; n =2 × 10 3 , two-tailed t -test; Fig. 5 ); gene pairs in one organism tend to have similar 3DGD and CUFS to the orthologues in the second organism. The two mammals, which diverged more recently than the fungi, show a greater similarity in their genomic 3D architecture. It should be noted that orthologous genes tend to be more conserved, in terms of sequence and potentially function than other genes in the genome [46] . 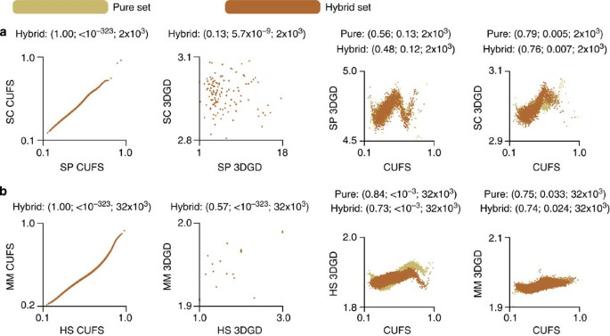Figure 5: Evolution of 3D genomic organization and function. The scatter plots in the figure comprise of a ‘pure’ set, containing data on both axes from the same organism; and a ‘hybrid’ set mixing data from two organisms (for example,S. cerevisiaeCUFS withS. pombe3DGD). The common organism for the two sets is denoted on they-axis (for example, SP 3DGD). Colours denote the source of thex-axis data (hybrid/pure). The first two plots in each panel show only the hybrid set, while the rest present both. Spearman’s rank correlation,Pvalues (two-tailedt-test for the first two plots, P3Dfor the other two) and the number of points is reported in parentheses above each plot in this order. All pure results show higher correlation than the hybrid ones. It is evident that there is a very strong conservation of CUFS, and a significant conservation of genomic organization. (a) Fungi evolution. (b) Mammalian evolution. Figure 5: Evolution of 3D genomic organization and function. The scatter plots in the figure comprise of a ‘pure’ set, containing data on both axes from the same organism; and a ‘hybrid’ set mixing data from two organisms (for example, S. cerevisiae CUFS with S. pombe 3DGD). The common organism for the two sets is denoted on the y -axis (for example, SP 3DGD). Colours denote the source of the x -axis data (hybrid/pure). The first two plots in each panel show only the hybrid set, while the rest present both. Spearman’s rank correlation, P values (two-tailed t -test for the first two plots, P 3D for the other two) and the number of points is reported in parentheses above each plot in this order. All pure results show higher correlation than the hybrid ones. It is evident that there is a very strong conservation of CUFS, and a significant conservation of genomic organization. ( a ) Fungi evolution. ( b ) Mammalian evolution. Full size image Importantly, similarity was conserved even when the distribution of codons in the respective orthologues had diverged (for example, r =0.53 between the CAI of genes in SC versus their CAI in SP based on the set of highly expressed SC genes). These results support the conjecture that both the relative 3D locations of genes and their CUFS are functionally important: While relatively large changes in codon bias in the two organisms have occurred, most functions of the genes that appear in both SC and SP are similar, and thus the within-organism CUFS and 3DGD in such genes is conserved in these two species. Adaptation of the spatial organization to genes’ function In evolution, organisms diverge and adapt to their environment, and thus gene function and genomic organization should evolve with them. If indeed function and 3D localization are strongly interconnected, we expect to be able to observe an evolutionary process between them, as the one property will constrain the diversification of the other. To test for such evolution for gene pairs, we compared the correlations obtained above to that of simulated ‘hybrids’ (for example, CUFS of SC versus 3DGD of SP and vice versa ), while focusing on genes that appear in both organisms (details in Methods). As can be seen in Fig. 5 , the correlations in the hybrid sets are lower than those observed for the original genomes. This result supports the conjecture that, even though the function of the analyzed orthologue families tends to be maintained, there is still an observed signal of adaptation of genes’ organization to their function, and that evolution tends to shape eukaryotic genomes in a way that maintains spatial clusters of genes with related functions. CUFS-3DGD correlation only partially explained by other nucleotide properties To further show that indeed codon distribution is the major explanation for the correlation between CUFS and 3DGD (rather than alternative properties related to the nucleotide distribution of genes or the genomic regions further away from them), we conducted a series of tests. First, we computed synCUFS on the first 200 codons after the start of each ORF (synCUFS-f0) to define a measure that is independent of gene length, unlike the complete-gene synCUFS that may be affected by gene length. We utilized this measure to perform a number of tests ( Fig. 6 , see also the Supplementary Methods ). In the first test, we show that the significant correlation for synCUFS is preserved in synCUFS-f0 for all organisms and P 3D is significant for almost all organisms, despite the decrease in the information it contains (SP: r =0.86, P <10 −323 , P 3D =0.022; n =2 × 10 3 ; SC: r =0.32, P <10 −323 , P 3D =0.226, n =2 × 10 3 ; AT: r =0.78; P <10 −323 ; P 3D =0.016; MM: r =0.93, P <10 −323 , P 3D =0.002, n =32 × 10 3 ; HS: r =0.87, P <10 −323 , P 3D <10 −3 , n =32 × 10 3 ). In the second test, we compared the correlations obtained for the two shifted reading frames (synCUFS-f1 and synCUFS-f2; Supplementary Fig. 7 ) and showed that they were lower on average (and specifically lower in three out of five organisms in frame 1, four out of five in frame 2) than the actual reading frame (synCUFS-f0; frame 1 average r =0.45 versus frame 2 r =0.43 versus real r =0.75). Since the shifted sequences are nearly identical to the ORF (only the reading frame is different), we expect some of the low-dimension signals (such as GC content and the distribution of pairs of nucleotides), as well as higher-dimension signals, to be partially retained. Thus, the fact that we still obtain a relatively high correlation is not surprising. The result teaches us that it is possible to partially infer the functional similarity of genes based on shifted ORFs, but that a larger amount of relevant information appears in the correct frame. In the third test, we computed synCUFS on random-genes (of length 200) constructed from sequences that lie adjacent to a gene’s ORF upstream or downstream of it without overlapping it (random-synCUFS), to show that the correlation decreases considerably and is deemed insignificant by P 3D when considering the random sequences (random 500 nt downstream average r =−0.16 versus random 500 nt upstream r =−0.11 versus real r =0.75; see Supplementary Note 3 on extreme values in the random scatter plots). In the fourth test, we compared again CUFS to two other components that are contained within CUFS: synCUFS, which measures the difference in the distribution of synonymous codons, and AAFS, which measures the only the difference in the distribution of amino acids. Again, we see varied results: CUFS is more strongly correlated than synCUFS in SC, mouse and human (SP: r =0.83; SC: r =0.33; AT: r =0.73; MM: r =0.95; HS: r =0.88; Supplementary Fig. 8 ), and is more strongly correlated than AAFS in all organisms but SC (SP: r =0.26; SC: r =0.72; AT: r =0.58; MM: r =0.80; HS: r =−0.09). This demonstrates that both synCUFS bias and amino acid bias contribute to the correlation between CUFS and 3DGD. Similar tests were performed for other measures of codon usage ( Supplementary Figs 9 and 10 ). 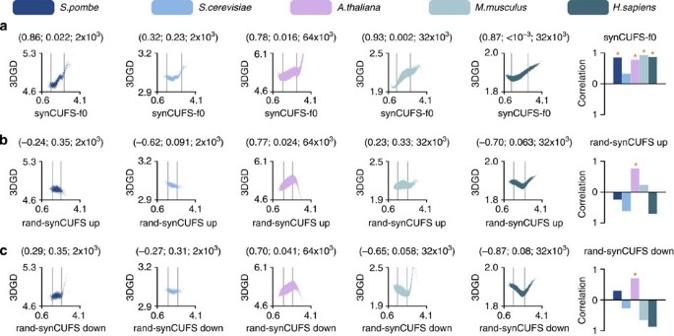Figure 6: Locality tests. (a) Scatter plots of 3D genomic distance (3DGD) versus synCUFS, computed over the first 200 codons of the reading frame (synCUFS-f0) for the five organisms. Spearman’s rank correlation, P3DPvalues and number of points are reported in parentheses above each plot in this order. Vertical markers denote the top/bottom 5% of values, so that 90% are contained within them. Bars denote Spearman’s rank correlation coefficient,Pvalues were computed using the cyclic chromosome shift model (P3D, 1,000 samples drawn); stars mark significant correlations (P3D<0.05). (b) Scatter plots of 3D genomic distance (3DGD) versus synCUFS, computed over random intergenic sequences 500 nt upstream of the ORF (rand-synCUFS up). (c) Scatter plots of 3D genomic distance (3DGD) versus synCUFS, computed over random intergenic sequences 500 nt downstream of the ORF (rand-synCUFS down). Figure 6: Locality tests. ( a ) Scatter plots of 3D genomic distance (3DGD) versus synCUFS, computed over the first 200 codons of the reading frame (synCUFS-f0) for the five organisms. Spearman’s rank correlation, P 3D P values and number of points are reported in parentheses above each plot in this order. Vertical markers denote the top/bottom 5% of values, so that 90% are contained within them. Bars denote Spearman’s rank correlation coefficient, P values were computed using the cyclic chromosome shift model (P 3D , 1,000 samples drawn); stars mark significant correlations (P 3D <0.05). ( b ) Scatter plots of 3D genomic distance (3DGD) versus synCUFS, computed over random intergenic sequences 500 nt upstream of the ORF (rand-synCUFS up). ( c ) Scatter plots of 3D genomic distance (3DGD) versus synCUFS, computed over random intergenic sequences 500 nt downstream of the ORF (rand-synCUFS down). Full size image CUFS correlates better with 3DGD than the genes’ GC content In SC, GC content was reported to be correlated with recombination frequency [47] , while crossover recombination sites were reported to be enriched in Hi-C contacts [20] . In addition, centromeres have been reported to be strongly co-localized [12] , and have also been characterized as having low GC content [48] . In mammals, GC content was shown to be related to co-localized active transcription domains in the chromosomes [6] , [11] , [16] . These reports may suggest that GC content similarity (GC Sim) between genes, which is a CUFS-related feature, should also have relatively high correlation with 3D gene genomic distance. Indeed, a high correlation between GC similarity and 3DGD has been observed. Specifically, GC similarity significantly correlated with 3D gene genomic distances in SC ( r =0.64; P <10 −323 ; P 3D =0.028; n =2 × 10 3 ), SP ( r =0.62; P <10 −323 ; P 3D =0.078; n =2 × 10 3 ) and to a higher degree in MM ( r =0.89; P <10 −323 ; P 3D <10 −3 ; n =32 × 10 3 ) and HS ( r =0.98; P <10 −323 ; P 3D <10 −3 ; n =32 × 10 3 ). It is worth noting, that in AT, where GC similarity was found to be weakly correlated with CUFS ( r =0.11; P <10 −323 ; n =64 × 10 3 ), it was also found to be weakly correlated with 3DGD ( r =−0.35; P <10 −323 ; P 3D =0.044; n =64 × 10 3 ). It is important to note that GC content, as defined in this work (computed over the ORF) is an aspect of CUFS and thus the two are expected to show the same trend. In addition, we show that the correlation with it cannot be explained by various experimental biases [6] , [20] , [49] (see below, and also the Supplementary Methods ). For instance, it is evident in Supplementary Fig. 11 that segment GC Sim (referring to HindIII restriction fragments in the Hi-C experiment) is less correlated with 3D distances than the GC content. In addition, the very high correlation reported here cannot be explained by the phenomena reported in the papers mentioned above [12] , [47] , [48] , and is probably related to additional explanations such as various aspects of gene expression regulation that are related to mRNA folding and GC content [28] , [50] , [51] . To establish that CUFS is correlated with 3D genomic distances independently of other dominant gene features ( Supplementary Fig. 12 ), particularly GC similarity, we show that the correlation is retained also when using only gene pairs with identical gene GC content (SP: r =0.66; P =9.2 × 10 −14 ; P 3D =0.105; n =100; SC: r =0.78; P =1.1 × 10 −21 ; P 3D =0.016; n =100; AT: r =0.76; P <10 −323 ; P 3D =0.025; n =3,200; MM: r =0.88; P <10 −323 ; P 3D =0.034; n =1,600; HS: r =−0.38; P <10 −323 ; P 3D =0.53; n =1,600), or identical segment GC content (see Methods; SP: r =0.49; P <2.5 × 10 −7 ; P 3D =0.169; n =100; SC: r =0.65; P =1.6 × 10 −13 ; P 3D =0.032; n =100; AT: r =0.78; P <10 −323 ; P 3D =0.017; n =3,200; MM: r =0.95; P <10 −323 ; P 3D <10 −3 ; n =1,600; HS: r =0.56; P <10 −323 ; P 3D <10 −3 ; n =1,600). Furthermore, we computed the partial correlations of each of the main gene features identified to be correlated with genomic distance, given all other features ( Supplementary Fig. 13 ), as well as Hi-C experimental biases. It is evident that CUFS attained the highest and most consistent partial correlation (highest mean, with a low cross organism variance; SP: r =0.76, P 3D <0.01; SC: r =0.56, P 3D <0.01; AT: r =0.56, P 3D =0.02; MM: r =0.95, P 3D <0.01; HS: r =0.80, P 3D =0.01), which is considerably higher than any GC-related feature. While the average partial correlation for CUFS is 0.73, all other average partial correlations are <0.38. Thus, the results support the conjecture that the correlation between CUFS and 3DGD is not only due to GC Sim or any other gene feature. In summary, two major fundamental conclusions can be derived from the results. First, we show that CUFS can serve as a proxy for gene function and expression patterns, and strongly correlates with 3DGD. CUB is known to be related to gene expression optimization [29] , mRNA folding stability, amino acid content and gene function [25] , [26] , [27] , [28] , [30] and may also be related to yet unknown molecular mechanisms in the eukaryotic cell. Thus, our analyses demonstrate that CUFS is a robust measure, insensitive to a particular experimental protocol, which can be used for computing functional similarity among genes in future systems biology and genomic studies. We would like to reiterate that our definition of CUFS is not related only to translation elongation, but to all aspects of gene expression and function that are encoded in the ORF. Thus, it is possible that extended functions of higher complexity based on codon and nucleotide distribution (for example, codon pairs and k-mers) may provide an even more comprehensive description of functional similarity, and a better explanation of 3D genomic organization of genes. Answers to this topic are deferred to future studies. Second, the results reported in this study also support the conjecture that there is a very high level of global genomic organization in several eukaryotes such as SC, SP, AT, MM and HS, which is 3D in nature. Thus, the location of genes across the eukaryotic genome, and the way that they are packaged in 3D space is far from being random and can be explained by their function and expression pattern. These conclusions encourage further experimental and computational studies to infer and understand the spatial organization of chromatin at a high resolution. To conclude, we briefly demonstrate that the associations reported in this study can be obtained via other representations of 3D genomic organization. We were able to reproduce the significant positive correlation of CUFS with 3D model distance in two previously published whole-genome models (SC: r =0.60; P <10 −323 ; n =2 × 10 3 ; SP: r =0.36; P <10 −323 ; n =2 × 10 3 ; Supplementary Fig. 14 ). The two models were generated by solving a beads-on-a-string problem under constraints obtained from Hi-C experiments [12] , [13] . Furthermore, a comparison of the median CUFS between sets of pairs of genes with the top/bottom 2% of Hi-C scores showed a significant decrease in CUFS for pairs with high Hi-C reads (that is, having high physical proximity; Wilcoxon rank-sum test: SP: P =5 × 10 −11 ; SC: P <10 −323 ; AT: P <10 −323 ; MM: P <10 −323 ; HS: P <10 −323 ; Supplementary Fig. 14 , details in the Supplementary Methods ). Thus, the last result is based on minimal modelling assumptions and confirms our previous results. Both aforementioned conclusions regarding functional similarity and genomic organization can be employed for improving the approaches for inferring the 3D organization of genomes, for developing accurate models of genomic evolution and organization and for studying/understanding gene function, expression and evolution. Hi-C data The available contact maps for the five organisms are the output of various closely related high-throughput experimental protocols. All protocols were derived and adapted from 3C ref. 10 , and are regarded in this work—for the sake of simplicity—as Hi-C methods. Supplementary Table 1 summarizes the data set chosen for each organism. It can be seen that some parameters vary between data sets. Most importantly, the given resolution for each data set is different with a variability of up to 2 orders of magnitude (compare SP and HS). While all the experiments were done using HindIII restriction enzymes to produce DNA segments that make up the basic unit of raw contact maps, four out of five data sets employed constant size bins to collect the measurements to improve the signal to noise ratio [11] , [13] , [16] , [17] . The size of bins determines the resolution of the data set in these cases. In addition, three out of the five data sets were corrected to minimize experimental biases [13] , [16] , [17] . The data set for SC was further filtered to include a selected portion of the contact map that passed 1%-FDR (ref. 12 ). All data sets went through additional post processing, as noted in Supplementary Table 1 . We completed the processing of the provided data by choosing a post process that minimizes biases in the data and maximizes its significance. We employed an iterative correction process based on ref. 52 , similar to the one used for the mouse data set (for details, see the Supplementary Methods ). Cis maps were then normalized using the expected Hi-C read by genomic distance. Furthermore, we kept only the top percentage of significant Hi-C measurements after the correction (see Supplementary Table 1 ). Cis maps (intrachromosomal) and trans maps (interchromosomal) were filtered separately to insure that both types of interactions are represented properly. The filter threshold was chosen according to genome size and Hi-C map density. The above treatment aims at reducing the differences between data sets, before proceeding to a general, non-specific protocol of analysis. While all results in this work are in general agreement between organisms, some of the diversity between organisms (for example, different levels of correlation) may be attributed to the differences in the protocols, their execution and inherent biases, as well as the preparation of the data. For instance, the HS map was measured on cycling cells, while the data set for MM was measured on cells in the same phase of the cell cycle (G1-arrested cells) [16] . Genome sequence Fungal and plant genome sequences were obtained from NCBI (SC S288c strand and SP 972h strand, AT TAIR10), which include 5,123 protein-coding SP genes ( http://www.pombase.org/status/statistics , mRNA-protein_coding), 5,888 SC genes ( http://www.ncbi.nlm.nih.gov/bioproject/PRJNA128 , Protein Sequences) and 27,191 AT genes ( ftp://ftp.arabidopsis.org/home/tair/Genes/TAIR10_genome_release/README_TAIR10.txt , see also Supplementary Table 2 ). We located all the HindIII restriction sites in SC and updated the coordinates of the SC Hi-C map. We used the NCBI protein tables for the ORF sequences. Since the Hi-C contact maps for mammals were based on the mm9/hg18 versions of the genomes, we used the UCSC table browser tool [53] to generate gene tables for HS hg18/hg19 genomes and MM mm9/mm10 genomes. In our analyses, for example, in HS, we used the set of genes that is shared by the two tables—hg18 and hg19. This enabled us to use updated gene sequences for most of the known protein-coding genes (see Supplementary Table 2 ). Genome sequences for hg19/mm10 were obtained from NCBI. 3D genomic distance We utilized the Hi-C contact maps to construct graph/network representations of the spatial organization of the genome. The high resolution of the chosen contact maps allowed us to investigate the 3D structure in single protein-coding gene resolution by representing each gene as a node. In the case of mammals, each node represents all the possible products by alternative splicing of this gene. Binned chromosome interactions from the contact maps were transformed into gene-gene interactions. We mapped every gene to its closest Hi-C bin according to the distance between their centre coordinates. Each bin’s contacts with all others were assigned to its mapped genes. We tried several criterions for mapping the data from Hi-C bins to genes to choose the least biased one, including: all overlapping bins per gene; maximum-overlap of bin per gene (as in ref. 20 ); maximum-overlap of gene per bin and weighted mapping that is proportional to the overlap between bin and gene. We were able to reproduce our main results with all the aforementioned methods. Since Hi-C maps were already filtered to include only the most significant interactions (see previous sections), we used binary graph edges (1/0) to depict interactions between genes. Chromosomes backbone edges between adjacent genes on the same chromosome were added to this graph, so that all neighbouring genes are at distance 1 from each other. Graph distances between all pairs of genes were computed according to the shortest path between them and were measured in hops. This setting allowed us to work in single-gene resolution, compute the distance between any given pair of genes and incorporate both interchromosomal and intrachromosomal measurements (some of the previous studies used only one of the two kinds). Codon usage frequency similarity Codon usage frequency vectors were computed by counting all appearances n i of a codon i in the ORF, and dividing by the total codon count. It can be seen that this vector combines both the CUB and amino acid usage bias, because the frequency of each codon is normalized with respect to all other codons, not only synonymous codons for the same amino acid. We used the average frequency vector for genes with a number of alternatively spliced transcripts. synCUFS frequency vectors were computed as follows: Where the number of observed codons n i is normalized by the sum of all synonymous codons coding for the same amino acid or stop codon rather than all other codons. AAF vectors were computed as follows: Where n i is the number of counted occurrences of amino acid i in the ORF. The CUFS between genes was computed using the Endres–Schindelin metric [23] for probability distributions. Given the frequency vectors of a pair of genes p and q , the CUF distance/similarity between them is given by: Where d KL is the Kullback–Leibler divergence—a popular information gain measure, that is non-symmetric and does not satisfy metric properties [54] . Its use in this context, however, satisfies all required properties for a metric. It also bears a similarity to the Jensen–Shannon divergence. AAFS and synCUFS were computed using the same metric. CUB indices We computed the CAI [42] , tAI [29] , bcENC [43] —which is an improved variant of the effective number of codons [55] , CDC [44] and the RCB [45] index according to the cited papers. The reference set for CAI was selected according to the available protein abundance data [56] (see also the Supplementary Methods ), by taking the top 100 expressed genes. The background nucleotide composition for CDC was estimated from the entire coding sequence of the genome, while for bcENC and RCB it was estimated from the ORF of each gene separately. PPI graph We used a number of PPI databases [57] , [58] , [59] , [60] , [61] , [62] to construct an undirected PPI network for the five organisms, and used the shortest path on the graph to define the PPI graph distance between each pair of genes. Disconnected pairs were assigned with a finite scalar (255) to include them in the average graph distance calculation, so that the PPI distance value for a set of gene pairs ranges from 1 (adjacent neighbours set) to 255 (completely disconnected set). (See also the Supplementary Methods ). GO term distance We used the full GO [63] annotations provided for the five organisms [64] , [65] , [66] , [67] , [68] , and mapped them onto the generic slim ontology definitions provided by GOC, except in the case of AT where the plant slim ontology definitions were used. The distance between a pair of GO terms was defined to be the sum of the distances of the two terms on the GO graph from their least common ancestor. The distance for a pair of genes was computed by averaging the GO term distance between all their terms in the biological process ontology. Other similarities Distance for other measures, such as GC content and gene length, which are given as scalars for each gene, were computed as normalized distance: Scalars given for different splice alternatives (such as GC and length) were averaged per gene before computing the distance. Correlation Correlation was computed using a defined number of bins n according to the test of interest. Binning was conducted as follows. The measure in question, for example, CUFS, was computed for all gene pairs, then n bins of equal size of CUFS values were set, dividing all pairs. The mean CUFS and mean 3D distance were computed for each bin; finally, Spearman’s rho was computed between all CUFS/3D distance bins. Supplementary Figure 5 presents the resultant correlation with CUFS/3D distance of different features for various bin sizes. The chosen number of bins for AT ( n =64 × 10 3 ) and mammals ( n =32 × 10 3 ) was larger than that for fungi ( n =2 × 10 3 ) to account for their larger genome (measured in number of protein-coding genes, or nodes on the genomic graph). We preferred binning the pair of variables being tested for correlation according to the variable with the widest range of values (closest to being continuous) to improve statistical accuracy. When binning integer values, specifically the 3DGD, we found that the distribution of 3D distances led to numerous bins holding the same distance value. For this reason, the variable tested against 3D distance was the one defining the bins in all cases; when testing a variable against CUFS, bins were defined by CUFS, which is a continuous distance measure. In two cases, however, we binned the variables according to 3D distance (see the Supplementary Methods ). P value computation Statistical significance of the results was verified against an empirical null model—cyclic chromosome shift ( Fig. 3a ). We draw from this model by randomly shifting the location of all genes on their respected chromosomes. The underlying null hypothesis is that the co-localization of specific gene sets of interest is not driven by the chromosome spatial conformation. In practice, drawing from the model is done by shifting the labels of all nodes while leaving the edges unmodified. P values were calculated by drawing 1,000 samples (random genome configurations) from the model and estimating the distribution of correlation coefficients ( Fig. 3b,c ), according to: Where 1 {} is the indicator function, r i is the random correlation coefficient obtained and r exp the observed correlation coefficient in the experiment. The cyclic chromosome shift model we used, beside its inherent logic, is the most conservative of the ones we tested, including: two-tailed t -test for Spearman’s correlation; degree-preserving rewiring of the graphs; random sampling of gene sets/gene pairs and cyclic genome shift, which is a whole-genome cyclic shift, allowing genes to rotate and move between chromosomes freely. Evolution and conservation For the fungal evolution results, we used the manually curated orthologues database at PomBase [69] , containing 3,367 orthologue families. For mammalian evolution, we used the MGI report of Human and Mouse Homology Classes sorted by HomoloGene ID [67] (file: HOM_MouseHuman Sequence.rpt) containing 15,832 orthologue families. We utilized the orthologue families to transform the CUFS/3D distance matrices, so that the transformed Co-CUFS for a pair of genes is the average CUFS between their corresponding orthologues in the co-organism. So that, given a distance matrix D B in organism B, the orthologous-transformed matrix in organism A is given by: where O j is the set of orthologous genes in organism B corresponding to gene j in organism A. We then followed the correlation procedure, but considered only genes with identified orthologues in both species. The regular test consisted of computing the correlation of, for example, CUFS for orthologue sets of genes in organism X with the 3DGD in X. The obtained correlation was different than that computed for all possible genes following the use of only a subset of these. The hybrid test consisted of computing the correlation of, for example, the transformed Co-CUFS matrix for organism Y with the 3DGD in organism X. The conservation of hybrid sets of CUFS versus CUFS and 3DGD versus 3DGD was computed in the same manner. HindIII segment properties For control purposes, we located all the possible HindIII segments (cut site AAGCTT) in the genomes and computed their length as well as segment GC content (in a window of 200 nt upstream of the cut site, as in ref. 6 ). We discarded HindIII segments larger than 100,000 nt. The average segment GC content/length was computed for each Hi-C bin. Nodes (genes) on the graph were then assigned with segment length/GC content according to the Hi-C bin they were assigned when constructing the 3D genomic graph. When testing for identical node pairs, we included the 5% of pairs with the closest property value (for example, segment GC content), and binned them according to CUFS using 5% of the number of bins to account for the reduction in the amount of data. Partial correlations We demonstrated that CUFS is strongly correlated with many other variables ( Supplementary Fig. 1 ). In the partial correlations test, we computed the partial correlation for nine features of the graph nodes, each correlation given the other eight. To this end, all variables were binned according to the 3D distances so that they can be compared (using min-variance binning, see Supplementary Methods ). We used Spearman’s correlation. How to cite this article: Diament, A. et al. Three-dimensional eukaryotic genomic organization is strongly correlated with codon usage expression and function. Nat. Commun. 5:5876 doi: 10.1038/ncomms6876 (2014).